Hidden two-qubit dynamics of a four-level Josephson circuit Multi-level control of quantum coherence exponentially reduces communication and computation resources required for a variety of applications of quantum information science. However, it also introduces complex dynamics to be understood and controlled. These dynamics can be simplified and made intuitive by employing group theory to visualize certain four-level dynamics in a ‘Bell frame’ comprising an effective pair of uncoupled two-level qubits. We demonstrate control of a Josephson phase qudit with a single multi-tone excitation, achieving successive population inversions between the first and third levels and highlighting constraints imposed by the two-qubit representation. Furthermore, the finite anharmonicity of our system results in a rich dynamical evolution, where the two Bell-frame qubits undergo entangling–disentangling oscillations in time, explained by a Cartan gate decomposition representation. The Bell frame constitutes a promising tool for control of multi-level quantum systems, providing an intuitive clarity to complex dynamics. Quantum information science, where quantum dynamics meets information theory [1] , [2] , [3] , promises to revolutionize critical aspects of our ability to compute and communicate. The theoretical framework of quantum information calls for controlled quantum machinery, typically based on two-level transitions, coherence and readout, a.k.a. qubits. Many physical systems commonly used as qubits, such as trapped ions [4] , [5] and superconducting circuits [6] , [7] , are in reality multi-level systems whose dynamics are manually limited by researchers to two levels to preserve simplicity and fidelity. Such systems can easily be employed as multi-level qudits by accessing additional levels, allowing a significant reduction of the resources and gates required for a variety of quantum information applications [8] , [9] , [10] , yet also introducing a complex multi-level problem. The usefulness and popularity of multi-level qudits are limited by a dearth of theoretical methods for understanding and controlling their dynamics. In this paper we study the reduction of four-level dynamics to a pair of two-level qubits, providing a familiar geometric representation for a multi-level system. The recently proposed control scheme of Pythagorean coupling [11] , which introduces a family of solutions for successive complete inversions in a four-level system, is a suitable springboard for this purpose. Continuous group theory plays a central role in quantum dynamical systems, providing powerful tools to describe their evolution in terms of quantum states and control operations [12] , [13] , [14] , [15] . For quantum information, the relevant groups are the SU(2) and SU(4) symmetry groups, which serve as building blocks of a universal quantum computer. The dynamics of a two-level quantum system is described by the SU(2) group, which is represented with 2 by 2 unitary matrices. Systems possessing this symmetry lend themselves to straightforward geometric interpretation as a Bloch vector, where a normalized quantum state is mapped to a point on a sphere. This picture is extremely useful in quantum information, as single-qubit gates rotate the Bloch vector and decoherence has the effect of pulling it towards the z -axis [16] . While SU(2) dynamics are used for local qubit manipulation, SU(4) dynamics allow nonlocal manipulation of qubit pairs. With the machinery of Cartan decomposition [17] , the SU(4) group can be factored into local qubit rotations and a non-local two-qubit entanglement operation. As the SU(4) group also describes a four-level quantum system, such a decomposition allows the dynamics of a four-level qudit to be mapped onto and subsequently visualized by a pair of coupled two-level qubits. Anticipating local control of the qubit pair as described below, we relate the ‘Lab frame’ qudit states {|0›, |1›, |2›, |3›} and the ‘Bell frame’ two-qubit states {|00›, |01›, |10›, |11›} through the following transformation: A unique subgroup of the full SU(4) is the SO(4), the Euclidean four-dimensional rotation symmetry, defined by six independent parameters. The useful identity SO(4) ≅ SU(2) ⊗ SU(2) implies one-to-one mapping of the four-dimensional rotational dynamics to those of an uncoupled pair of Bloch vectors [11] . In other words, if the dynamics of a four-level qudit was limited to SO(4), the dynamics in the Bell frame would be comprised solely of single-qubit rotations without inter-qubit coupling (see Fig. 1 ). 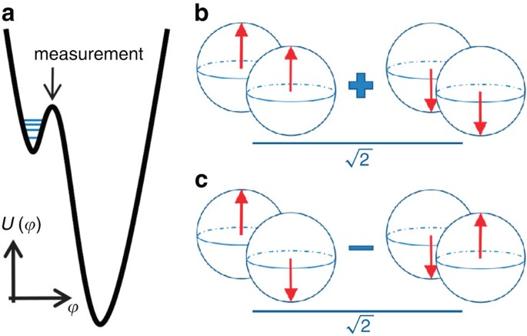Figure 1: The four-level Lab-frame system and the two-qubit Bell-frame system. (a) The phaseϕof a flux-biased superconducting Josephson qudit is localized in a shallow potential well, giving rise to a number of anharmonically spaced energy levels. The multi-level qudit state is measured by lowering the potential barrier, causing the phase to tunnel out of the shallow well. (b) The states of a four-level qudit can be mapped onto a pair of two-level qubits. For example, the two-qubit statedepicted here by the Bloch spheres corresponds to the state |0› of the physical Lab-frame qudit. SO(4) rotations in the Lab frame factor exactly into local rotations of the Bell-frame qubits, while SU(4) rotations couple them together. (c) The depicted two-qubit statecorresponds to the state |2› in the Lab frame. The Pythagorean coupling scheme achieves population inversion between the Lab-frame states |0› and |2› by synchronizing rotations of the Bell-frame qubits. Figure 1: The four-level Lab-frame system and the two-qubit Bell-frame system. ( a ) The phase ϕ of a flux-biased superconducting Josephson qudit is localized in a shallow potential well, giving rise to a number of anharmonically spaced energy levels. The multi-level qudit state is measured by lowering the potential barrier, causing the phase to tunnel out of the shallow well. ( b ) The states of a four-level qudit can be mapped onto a pair of two-level qubits. For example, the two-qubit state depicted here by the Bloch spheres corresponds to the state |0› of the physical Lab-frame qudit. SO(4) rotations in the Lab frame factor exactly into local rotations of the Bell-frame qubits, while SU(4) rotations couple them together. ( c ) The depicted two-qubit state corresponds to the state |2› in the Lab frame. The Pythagorean coupling scheme achieves population inversion between the Lab-frame states |0› and |2› by synchronizing rotations of the Bell-frame qubits. Full size image We first note that a Hamiltonian generating SO(4) dynamics is , which is readily realized in the laboratory on a system with a ladder-type level configuration. In the theory of Pythagorean coupling [11] , this Hamiltonian is shown to cause complete population transfer between |0› and |2› in the Lab frame by rotating the state into the state in the Bell frame, contingent on the amplitudes ( V 01 , V 12 , V 23 ) being proportional to a primitive Pythagorean triple: for two odd integers p and q , the set is a primitive Pythagorean triple, so called because c 2 = a 2 + b 2 and the three elements do not possess a common divisor [18] . This solution for a four-level system stands in striking contrast to the resonant two-level problem, where complete population transfer is achievable for any coupling strength. With Pythagorean coupling, complete population transfer to the third level is attained when both Bell-frame qubits simultaneously complete an odd number of half-rotations, which is equivalent to p and q obeying the constraint for m , n ε Z . Here we experimentally show the effect on four-level dynamics of this rationality condition, which is in essence the fingerprint of the two-qubit picture. Moreover, we show that our experimental system, based on the flux-biased Josephson phase qudit, not only offers an elegant and useful way for exploiting detunings and decoherences, but also allows exploring the strongly interacting regime. Harnessing the anharmonicity of the physical qudit thus opens a gateway for optimal control in multilevel circuits. Experimental demonstration of Pythagorean coupling Our four-level quantum system is a flux-biased Josephson phase circuit [19] . We sweep two numbers, p and q , in the range [0, 2] and for each pair generate the corresponding Pythagorean triple. We then multiply the Pythagorean triple by a Rabi frequency Ω /2 π =47.62 MHz to obtain the amplitudes ( V 01 , V 12 , V 23 )= ħΩ × ( c , a , b ) and synthesize a three-tone pulse , where ħω i −1, i is the energy spacing between levels i and j and the denominators serve as harmonic-approximate corrections for the stronger coupling of the radiation to higher oscillator modes. The drive produces the Hamiltonian . Each coupling term includes off-resonant terms (see Supplementary Note 1 ). In the rotating wave approximation, valid at low drive amplitudes or, alternatively, for large anharmonicity, the Hamiltonian reduces to the form of H A . In such a circuit, related SU(2)-like controls have been demonstrated by emulating larger spin-states [20] . Pythagorean coupling generalizes this control to a four-level system, with two separate oscillation frequencies and subsequent rich dynamics. The Bell-frame approach can also be viewed as an analogue simulation of any coupled two-qubit control [21] . For each pair of ( p, q ) values, we initially apply the corresponding three-tone pulse for a duration of 60 ns and measure the populations of the four qudit states. 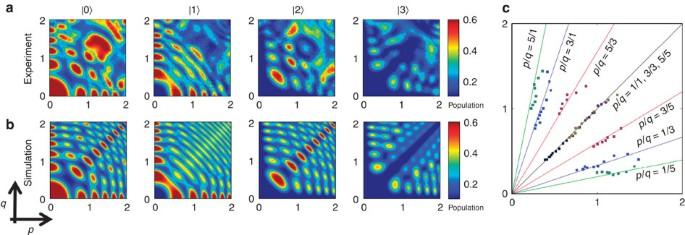Figure 2: Pythagorean dynamics in the Lab frame. (a) Experimental data taken after a 60 ns three-tone pulse. Axes correspond to (p, q) values used to generate a primitive Pythagorean triple, which is multiplied by a Rabi frequency to produce three coupling amplitudes. Excitation peaks of the third level appear when the two Bell-frame qubits simultaneously complete an odd number of half-rotations. (b) Simulation with ideal (infinite) qudit anharmonicity. The dynamics factor into SU(2)⊗SU(2) everywhere on thepqplane, producing a regular pattern of third-level excitation peaks. The deviation of the experimental results from ideal Pythagorean dynamics sufficiently far from the origin of thepqplane is attributed to the finite anharmonicity, and is probed by the higher drive amplitudes. (c) Third-level excitation peaks in thepqplane at different times. Eachp/qratio is characteristic of a particular excitation peak and is preserved over time. Peaks are measured at 7 ns increments and move towards the origin over time. The constraint of each peak to a straight line in thepqplane is the hallmark of SO(4) dynamics and is the Lab-frame expression of the synchronization of the Bell-frame qubits necessary for third-level excitation. Figure 2a shows the results in what we call the pq plane, where the axes correspond to the ( p, q ) values used to generate the Pythagorean triple. We observe nine distinct third-level excitation peaks with p / q ratios of 1/1, 1/3, 1/5, 3/1, 3/3, 3/5, 5/1, 5/3, 5/5 and obtain a maximum excitation of 56%. Figure 2: Pythagorean dynamics in the Lab frame. ( a ) Experimental data taken after a 60 ns three-tone pulse. Axes correspond to ( p, q ) values used to generate a primitive Pythagorean triple, which is multiplied by a Rabi frequency to produce three coupling amplitudes. Excitation peaks of the third level appear when the two Bell-frame qubits simultaneously complete an odd number of half-rotations. ( b ) Simulation with ideal (infinite) qudit anharmonicity. The dynamics factor into SU(2) ⊗ SU(2) everywhere on the pq plane, producing a regular pattern of third-level excitation peaks. The deviation of the experimental results from ideal Pythagorean dynamics sufficiently far from the origin of the pq plane is attributed to the finite anharmonicity, and is probed by the higher drive amplitudes. ( c ) Third-level excitation peaks in the pq plane at different times. Each p/q ratio is characteristic of a particular excitation peak and is preserved over time. Peaks are measured at 7 ns increments and move towards the origin over time. The constraint of each peak to a straight line in the pq plane is the hallmark of SO(4) dynamics and is the Lab-frame expression of the synchronization of the Bell-frame qubits necessary for third-level excitation. Full size image Figure 2b shows simulation using the Hamiltonian H A and decoherence assuming a Markovian noise source. Simulation and experiment agree very well for p , q ≪ 1.5 but begin to differ farther from the origin of the pq plane, where ( p, q ) values correspond to large drive amplitudes. We postpone discussion of this issue for the moment, and note that numerical simulation using the Hamiltonian H B fits the data remarkably well, reproducing even minor features both in the pq plane as well as in time-domain measurements (see Supplementary Figs 1,2 ). Bell-frame constraints on Lab-frame dynamics In the resonant two-level Rabi problem, changing the duration of the drive is equivalent to changing its amplitude; this is the well-known area theorem [16] . Similarly, as each point in the pq plane corresponds to a set of drive amplitudes, changing the pulse duration results in the excitation peaks of Fig. 2a appearing at different ( p, q ) values. However, optimal population transfer between the first and third states always requires a rational value of p/q , as this is a simple consequence of the dynamics in the Bell frame. To confirm that our qudit obeys this constraint, we sweep the pulse duration in the range 14–98 ns at intervals of 7 ns and measure the third-level population in the pq plane at each step. Figure 2c shows the locations of nine excitation peaks at different times as they move through the pq plane, each maintaining its characteristic value of the ratio p/q . This result showcases the physical importance and intuitive clarity of the Bell-frame dynamics, in contrast to the inherent complexity of multi-level dynamics. SO(4)-SU(4) crossover The difference between measurement and simulation shown in Fig. 2a,b is explained by noting that the Hamiltonian H B in the rotating wave approximation reduces to H A only in the limit of large anharmonicity. In the case of finite anharmonicity the off-resonant terms survive into the rotating frame. In this case, H B in the rotating frame can be written as the sum of H A and another matrix containing detuned coupling terms (see Supplementary Note 1 ). The latter operator takes the dynamics out of SO(4) into the full SU(4) dynamical space. As the identity SO(4) ≅ SU(2) ⊗ SU(2) is central to the theory of Pythagorean coupling, this symmetry is of the essence. As the coupling amplitudes grow large the off-resonant correction to H A becomes significant and so does the deviation of the qudit dynamics from SO(4) rotations. The experimental crossover from SO(4) to SU(4) dynamics is quantified by conducting a high-resolution measurement of the time-domain dynamics of the qudit population along the diagonal of the pq plane, sweeping the duration of the three-tone pulse in the range 1–200 ns ( Fig. 3a ). At lower amplitudes the excitation peaks of the |2› state behave as predicted by Pythagorean coupling theory. At higher amplitudes we observe a chevron pattern, which is readily understood in the Bell frame where SU(4) dynamics are mapped to single-qubit rotations with the addition of inter-qubit coupling. This coupling term changes the qubit resonance frequencies, thus affecting their respective detunings and Rabi oscillations. As the Bell-frame qubits are brought into resonance with their effective drives, their oscillation frequency decreases, manifesting as the chevron peak in the Lab-frame population. 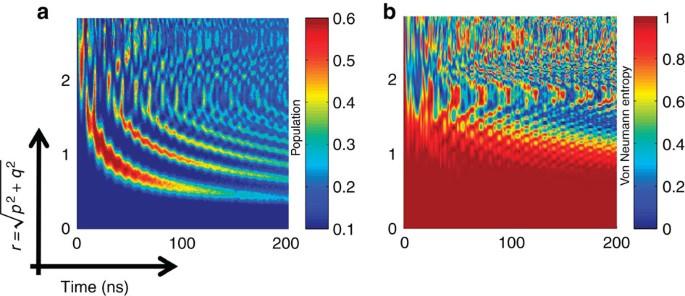Figure 3: Impact of finite anharmonicity on Bell-frame dynamics. The transition from SU(4) to SO(4) dynamics is measured by scanning (vertical) along the diagonal (p=q) of the pq plane (with a distance) and sweeping (horizontal) the duration of the three-tone pulse in the range 1–200 ns. (a) Population of the third qudit level. At low amplitudes excitation peaks move towards the origin so that, consistent with Pythagorean dynamics. At high amplitudes the dynamics transition from SO(4) to SU(4) because of the finite qudit anharmonicity. The larger group SU(4) does not factor into SU(2)⊗SU(2), but rather includes a term that couples together the Bell-frame qubits. The coupling terms shift their respective resonance frequencies, resulting in the chevron pattern. (b) Calculated von Neumann entanglement entropy of the Bell-frame qubits using the relationS= −Tr(ρAlog2ρA), whereρAis the reduced density matrix of one of the Bell-frame qubits. For low drive amplitudes where the dynamics factor into SU(2)⊗SU(2) the entanglement entropy is constant and maximum. The coupling terms become visible at high drive amplitudes and induce disentanglement–entanglement oscillations in the time domain. Figure 3: Impact of finite anharmonicity on Bell-frame dynamics. The transition from SU(4) to SO(4) dynamics is measured by scanning (vertical) along the diagonal ( p=q ) of the pq plane (with a distance ) and sweeping (horizontal) the duration of the three-tone pulse in the range 1–200 ns. ( a ) Population of the third qudit level. At low amplitudes excitation peaks move towards the origin so that , consistent with Pythagorean dynamics. At high amplitudes the dynamics transition from SO(4) to SU(4) because of the finite qudit anharmonicity. The larger group SU(4) does not factor into SU(2) ⊗ SU(2), but rather includes a term that couples together the Bell-frame qubits. The coupling terms shift their respective resonance frequencies, resulting in the chevron pattern. ( b ) Calculated von Neumann entanglement entropy of the Bell-frame qubits using the relation S = −Tr( ρ A log 2 ρ A ), where ρ A is the reduced density matrix of one of the Bell-frame qubits. For low drive amplitudes where the dynamics factor into SU(2) ⊗ SU(2) the entanglement entropy is constant and maximum. The coupling terms become visible at high drive amplitudes and induce disentanglement–entanglement oscillations in the time domain. Full size image This effect can be quantified by the bipartite entanglement in the Bell frame. Bipartite entanglement is parameterized by the von Neumann entropy, defined as S = −Tr( ρ A log 2 ρ A ), where ρ A is the reduced density matrix of one qubit [22] . Figure 3b shows the von Neumann entropy calculated from the Hamiltonian H B , ignoring decoherence to emphasize the point of interest. As the Lab-frame ground state corresponds to a maximally entangled state in the Bell frame, the von Neumann entropy attains its maximum value of unity. SO(4) operations do not affect the entanglement in the Bell frame, and accordingly for sufficiently low drive amplitudes the entropy retains its maximum value over time. In contrast, for large drive amplitudes the Bell-frame qubits are subjected to successive disentanglements and entanglements due to the component of the control (see Supplementary Note 2 ), resulting in disruption of the Pythagorean dynamics. In conclusion, we study the Bell-frame dynamics of a four-level system and demonstrate the first experimental implementation of a new coupling scheme—Pythagorean coupling, achieving population inversion between the ground state and the third state of a Josephson phase qudit with a single three-tone pulse. We obtain a peak third-level excitation of 56% consistent with simulation and qudit decoherence. The Bell-frame and Pythagorean dynamics apply to any generic four-level system, including longer coherence-time qubit circuits, such as the transmon/Xmon [23] , and the phase qudit was chosen for this work due to its highly convenient single-shot multi-level readout. Excitation of the third level depends strictly on the synchronization of the two Bloch vectors in the Bell frame, which is confirmed by following the excitation peaks through time in the pq plane. The finite anharmonicity of a physical qudit is shown to affect the dynamics by preventing their confinement to SO(4), causing oscillations in the Bell-frame bipartite entanglement entropy. The two-qubit Bell frame was introduced through a transformation that exactly factors the SO(4) group, thus helping uncover Pythagorean coupling as a method for population inversion, but its usefulness is far from exhausted. Properly detuning certain couplings may counterbalance the limiting effect of finite anharmonicity discussed in this work; alternatively, finite anharmonicity can be exploited as a feature. Non-Pythagorean Bell-frame dynamics are also highly useful, especially when using quantum systems with more controllable couplings than diamond- or ladder-type configurations. We expect the inherent complexity of multi-level dynamics to undergo more simplifications as the Bell frame is explored for coupling and control of larger systems. Josephson circuit operation The flux-biased Josephson phase qudit is magnetically coupled to an on-chip readout SQUID and cooled in a dilution refrigerator to a base temperature of ~20 mK. The phase of the Josephson junction is localized in a shallow potential well, giving rise to a number of anharmonic energy levels. The qudit state in the energy basis is measured via selective tunnelling of the phase to an adjacent deep well, which affects a detectable change in the SQUID critical current [24] . Measurements are averaged over ~1,000 repetitions to obtain probabilities. The qudit energy spectrum is controlled through a flux bias. The experiment was done with transition frequencies ω 01 /2 π =6.730 GHz, ω 12 /2 π =6.613 GHz and ω 23 /2 π =6.482 GHz. The relaxation and dephasing times of the |1› state were measured to be T 1 =230 ns and T 2 =110 ns without echo. The three-tone microwave pulse irradiating the qudit is synthesized by an IQ-mixer modulating a carrier frequency of 6.700 GHz. Other techniques are identical to those described in previous works on multi-level Josephson phase qudits [25] , [26] . How to cite this article: Svetitsky, E. et al. Hidden two-qubit dynamics of a four-level Josephson circuit. Nat. Commun. 5:5617 doi: 10.1038/ncomms6617 (2014).